Glucocerebrosidase mutations disrupt the lysosome and now the mitochondria 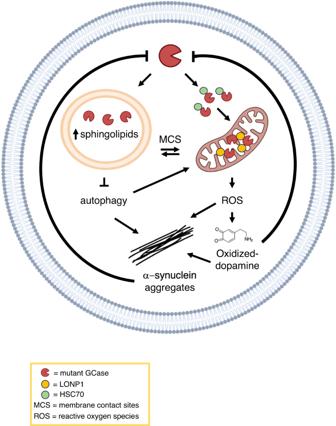Fig. 1: GCase exists in lysosomes and in mitochondria and plays a significant role in the pathological mechanisms of PD. Mutant GCase in lysosomes leads to elevated sphingolipid levels and hinders autophagic flux, resulting in the aggregation of a-syn into putatively toxic clusters. In turn, the accumulation of a-syn impairs GCase activity, initiating a detrimental cycle of cellular self-destruction. HSC70 imports GCase into mitochondria where it supports the proper functioning of mitochondrial complex I and maintains mitochondrial integrity. In this organelle, the protease LONP1 interacts with mutant GCase where it degrades it. Mutant GCase activity causes an increase in reactive oxygen species (ROS), leading to dopamine oxidation, increasing a-syn aggregation, and further impairment of GCase activity, creating a second pathological cycle. Additionally, autophagy deficiencies impair the elimination of a-syn and damaged mitochondria, leading to an additional rise in ROS levels. Furthermore, the lysosome and mitochondria are connected through membrane contact sites (MCS), facilitating the exchange of molecules, including toxic lipids and probably dysfunctional GCase. Black arrows indicate promotion of a mechanism and “T” indicates inhibition of the pathological loop. In conclusion, the mechanistic link between GBA1 variants and PD may lie in the interplay between GCase functions in the lysosome and mitochondria. GCase mutations that affect function in the lysosome lead to the intracellular accumulation of glycolipids, disrupting normal lysosomal function and autophagy, and leading to a-syn accumulation. Additionally, a-syn buildup impairs GCase activity, creating a self-perpetuating cycle of lysosomal dysfunction and a-syn accumulation, which may trap mitochondrial proteins in the cytosol, exacerbating both mitochondrial and lysosomal dysfunction. This could be investigated using similar proteomics approaches to Baden and colleagues, attempting to assess protein interactions in native conditions. GCase is also imported into the mitochondria via HSC70, where it promotes the integrity and function of mitochondrial CI. GCase mutations increase its interaction with LONP1, degrading GCase in mitochondria and promoting a-syn aggregation. Thus, mGCase increases ROS in mitochondria, oxidizing dopamine. In turn, the accumulation of oxidized dopamine-adducts further impairs GCase activity, creating a second cycle of GCase dysfunction (Fig. 1 ). The study by Baden et al. [16] further supports developing and testing GCase-based therapeutics in addition to the modulation of the mitochondrial quality control system for diseases with GCase dysfunction. We expect to observe novel brain penetrant GCase therapeutics, which in combination with other ongoing efforts such as dopamine replacement or stem cell approaches, may lead to important to urgently needed disease modifying therapies.